Detecting inertial effects with airborne matter-wave interferometry Inertial sensors relying on atom interferometry offer a breakthrough advance in a variety of applications, such as inertial navigation, gravimetry or ground- and space-based tests of fundamental physics. These instruments require a quiet environment to reach their performance and using them outside the laboratory remains a challenge. Here we report the first operation of an airborne matter-wave accelerometer set up aboard a 0 g plane and operating during the standard gravity (1 g ) and microgravity (0 g ) phases of the flight. At 1 g , the sensor can detect inertial effects more than 300 times weaker than the typical acceleration fluctuations of the aircraft. We describe the improvement of the interferometer sensitivity in 0 g , which reaches 2 x 10 -4 ms -2 / √Hz with our current setup. We finally discuss the extension of our method to airborne and spaceborne tests of the Universality of free fall with matter waves. Matter-wave inertial sensing relies on the capability of controlling the wave nature of matter to build an interferometer and accurately measure a phase difference [1] , [2] . As the particle associated to the matter wave senses inertial or gravitational effects, the interferometer represents an accurate inertial probe. In particular, atom interferometers (AIs) have benefited from the outstanding developments of laser-cooling techniques and reached accuracies comparable to those of inertial sensors based on optical interferometry. Because of their long-term stability, AIs offer a breakthrough advance in accelerometry, gyroscopy and gravimetry, for applications to inertial guidance [3] , geoid determinations [4] , geophysics [5] and metrology [6] . In addition, AIs are excellent candidates for laboratory-based tests of general relativity that could compete with the current tests that consider astronomical or macroscopic bodies [7] . For example, AIs may provide new answers to the question of whether the free-fall acceleration of a particle is universal, that is, independent of its internal composition and quantum properties. Although this principle—known as the Universality of free fall (UFF)—has been tested experimentally [8] , [9] to a few parts in 10 13 , various extensions to the current theoretical physics framework predict its violation (for a review of these theories, see ref. 10 ). It is thus important to test experimentally these theoretical models with different types of particles. AIs also open perspectives for further tests of general relativity such as the detection of gravitational waves [11] . All these fundamental tests may benefit from the long interrogation times accessible on microgravity platforms [7] , [12] , [13] , or in space [14] . Because of its high sensitivity, running an AI has required, until now, low-vibration and high-thermal stability environments that can only be found in dedicated ground or underground platforms. We report here the first operation of a matter-wave inertial sensor in an aircraft, both at 1 g and in microgravity (0 g ). Our matter-wave interferometer uses 87 Rb atoms and operates aboard the Novespace A300–0 g aircraft taking off from Bordeaux airport, France ( http://www.novespace.fr/ ). This plane carries out parabolic flights during which 22 s ballistic trajectories (0 g ) are followed by 2 min of standard gravity flight (1 g ). The AI measures the local acceleration of the aircraft with respect to the inertial frame attached to the interrogated atoms that are in free fall. In the first part of this communication, we describe the inertial measurements performed by our instrument and show how the matter-wave sensor achieves a resolution level more than 300 times below the plane-acceleration level. We present the general method that is used to operate the AI over a wide acceleration range and to reach such a resolution. In the second part, we demonstrate the first operation of a matter-wave inertial sensor in 0 g . Microgravity offers unique experimental conditions to carry out tests of fundamental physics. However, these experiments are conducted on platforms such as planes, sounding rockets or satellites, which are not perfectly free-falling, so that the residual craft vibrations might strongly limit the sensitivity of the tests. Overcoming this problem generally requires the simultaneous operation of two sensors to benefit from a common mode vibration noise rejection. For example, conducting a matter-wave UFF test implies the simultaneous interrogation of two different atomic species by two AIs measuring their acceleration difference [15] . In the present work, we investigate the 0 g operation of our one-species AI in a differential configuration to illustrate a vibration noise rejection. Our achievements (0 g operation and noise rejection) constitute major steps towards a 0 g -plane-based test of the UFF with matter waves at the 10 −11 level, and towards a space-based test [16] below 10 −15 . Such an experiment in space has been selected for the next medium-class mission in ESA's Cosmic Vision 2020–22 in the frame of the STE–QUEST project [17] (the report describing the STE–QUEST project is available in ref. 18 ). This paper presents the first airborne and microgravity operation of a matter-wave inertial sensor. We introduce a new and original method that allows to use the full resolution of an atom interferometer in the presence of high levels of vibration. We also show how high-precision tests of the weak equivalence principle may be conducted with differential atom interferometry. Description of the airborne atom interferometer Our experiment relies on the coherent manipulation of atomic quantum states using light pulses [19] , [20] . We use telecom-based laser sources that provide high-frequency stability and power in a compact and integrated setup [21] . Starting from a 87 Rb vapour, we load in 400 ms a cloud of about 3×10 7 atoms laser cooled down to 10 μK, and select the atoms in a magnetic field insensitive ( m F =0) Zeeman sublevel. We then apply a velocity selective Raman light pulse [22] carrying two counterpropagating laser fields so as to keep 10 6 atoms that enter the AI with a longitudinal velocity distribution corresponding to a temperature of 300 nK. The Raman laser beams are aligned along the plane wings direction ( Y axis, Fig. 1 ) and are retroreflected by a mirror attached to the aircraft structure and following its motion. The AI consists of a sequence of three successive Raman light pulses to split, redirect and recombine the atomic wavepackets ( Fig. 1d ). The acceleration measurement process can be pictured as marking successive positions of the free-falling atoms with the pair of Raman lasers, and the resulting atomic phase shift Φ is the difference between the phase of the two Raman lasers at the atom's successive classical positions, with respect to the retroreflecting mirror [23] . As the Raman beam phase simply relates to the distance between the atoms and the reference retroreflecting mirror, the AI provides a measurement of the relative mean acceleration a m of the mirror during the interferometer duration, along the Raman beam axis. The information at the output of the AI is a two-wave interference sinusoidal signal P = P 0 − A cos Φ , where P is the transition probability between the two 87 Rb ground states, and P 0 (resp. A ) is the offset (resp. the amplitude) of the interference fringes. This signal is modulated by the atomic phase shift Φ = a m × kT 2 , where k =2×2 π /780 nm is the Raman lasers effective wave vector and T is the time between the light pulses (see the first Methods subsection for the calculation of the phase shift). 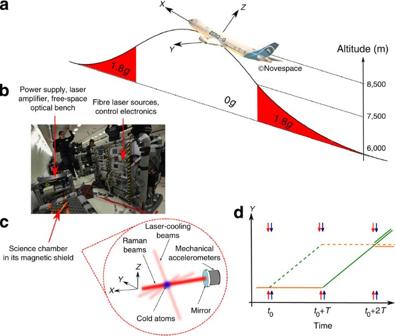Figure 1: Description of the experiment in the plane. (a) The parabolic manoeuvre consists of a 20 s pull-up hypergravity (1.8g) phase, the 22 s ballistic trajectory (0g) and a 20 s pull-out 1.8gphase. This manoeuvre is alternated with standard gravity (1g) phases of about 2 min and carried out 31 times by the pilots during the flight. (b) Picture of the experiment in the plane during a 0-g phase. (c) Zoom in the science chamber where the atoms are laser cooled and then interrogated by the Raman laser beams (red) that are collinear to the Y axis and retroreflected by a mirror (blue). (d) Space-time diagram of the AI consisting of three successive light pulses that split, reflect and recombine the two matter waves represented by the dashed and the solid lines. The blue and red arrows represent the two Raman laser beams. Figure 1: Description of the experiment in the plane. ( a ) The parabolic manoeuvre consists of a 20 s pull-up hypergravity (1.8 g ) phase, the 22 s ballistic trajectory (0 g ) and a 20 s pull-out 1.8 g phase. This manoeuvre is alternated with standard gravity (1 g ) phases of about 2 min and carried out 31 times by the pilots during the flight. ( b ) Picture of the experiment in the plane during a 0-g phase. ( c ) Zoom in the science chamber where the atoms are laser cooled and then interrogated by the Raman laser beams (red) that are collinear to the Y axis and retroreflected by a mirror (blue). ( d ) Space-time diagram of the AI consisting of three successive light pulses that split, reflect and recombine the two matter waves represented by the dashed and the solid lines. The blue and red arrows represent the two Raman laser beams. Full size image In the aircraft, the acceleration along Y ( Fig. 2a ) fluctuates over time by δa m ∼ 0.5 m s −2 (1 s.d. ), and is at least three orders of magnitude greater than the typical signal variations recorded by laboratory-based matter-wave inertial sensors. 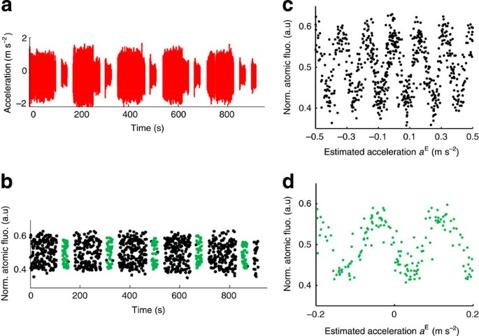Figure 2: AI revealing information on the plane acceleration. (a) Acceleration signal recorded by the MAs (red); the standard deviationδamof the acceleration signal is about 0.5 m s−2at 1gand 0.2 m s−2in 0g. (b) AI discrete measurements corresponding to the atomic fluorescence of the87Rb atoms in theF=2 state, normalized to the fluorescence of all the atoms; the total interrogation time is here 2T=3 ms. The black and green points correspond to the 1gand 0gphases, respectively; we have removed the 1.8gphases where the AI is not designed to operate. (c,d) Atomic measurements plotted versus the signal stemming from the MAs at 1g(c) and in 0g(d); the sinusoidal correlations show that the AI contains information on the acceleration of the plane. For this reason, the signal recorded by the AI first appears as random, as shown in Figure 2b . To quantify the information contained in the atomic measurements, we use mechanical accelerometers (MAs) fixed on the retroreflecting mirror and search for the correlation between the MAs and the AI [24] . We use the signal a MA ( t ) continuously recorded by the MAs to estimate the mean acceleration a E ( t i ) which is expected to be measured by the AI at time t i = iT c , with T c =500 ms being the experimental cycle time (see the first subsection in Methods). Plotting the atomic measurements P ( t i ) versus a E ( t i ) reveals clear sinusoidal correlations between the mechanical sensors and the AI, both at 1 g ( Fig. 2c ) and in 0 g ( Fig. 2d ). This demonstrates that the AI truly holds information on the mirror acceleration a m . We note that this result stands for the first demonstration of the operation of an atom accelerometer in an aircraft and in microgravity. Figure 2: AI revealing information on the plane acceleration. ( a ) Acceleration signal recorded by the MAs (red); the standard deviation δa m of the acceleration signal is about 0.5 m s −2 at 1 g and 0.2 m s −2 in 0 g . ( b ) AI discrete measurements corresponding to the atomic fluorescence of the 87 Rb atoms in the F =2 state, normalized to the fluorescence of all the atoms; the total interrogation time is here 2 T =3 ms. The black and green points correspond to the 1 g and 0 g phases, respectively; we have removed the 1.8 g phases where the AI is not designed to operate. ( c , d ) Atomic measurements plotted versus the signal stemming from the MAs at 1 g ( c ) and in 0 g ( d ); the sinusoidal correlations show that the AI contains information on the acceleration of the plane. Full size image Retrieving the plane acceleration with the AI resolution We now consider the application of our matter-wave sensor to precise measurements of the plane acceleration, by operating the AI beyond its linear range. For that purpose, we determine the AI acceleration response, defined by P AI ( a m )= P 0 − A cos( kT 2 × a m ), independently from the mechanical devices. We have developed a method (Methods) to estimate this response (that is, the parameters P 0 and A ), and the signal to noise ratio (SNR) of the interferometer, which determines the acceleration noise of the sensor, σ a =1/(SNR× kT 2 ). The knowledge of P 0 and A enables us to extract the acceleration a m ( t i ) from the atomic data P ( t i ) by inverting the model P AI ( a m ). In this way, the acceleration is known within the region where the interferometer model can be inverted unambiguously and corresponding to an acceleration interval of range a R = π / kT 2 . To obtain the total acceleration, we need the information on the reciprocity region ( n ( t i ) a R , ( n ( t i )+1) a R ) where the AI operates at measurement time t i , with n ( t i ) being the interference fringe number where the measurement point is located (Methods). To determine n ( t i ), we use the MAs which have a reciprocal response over a wide acceleration range. Thus, our instrument consists in a hybrid sensor that is able to measure large accelerations due to the mechanical devices, and able to reach a high resolution because of the atom accelerometer. 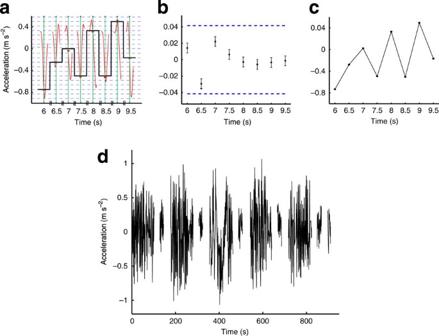Figure 3: High resolution measurement of the plane acceleration. (a) In red, signal recorded by the MAs in the time window (−2T,2T) around the measurement timesti=iTc(vertical green lines), withTc=500 ms and 2T=3 ms. The MAs signal has been filtered by the response function of the AI described in the Methods section, and the red points represent the value of the signal atti. This value determines the reciprocity region where the AI operates, delimited by two horizontal dashed lines. In this way, the MAs provide the coarse acceleration measurement (black step-like signal). (b) The AI is then used for the high-resolution measurement within its reciprocity region, bounded by the two blue dashed lines at ±aR/2, withaR=π/kT2≈0.087 m s−2. The error bars represent the noise of the atom accelerometer, which equals 0.0065 m s−2per shot in this example (SNR=4.3). (c) The total acceleration (am) is the sum of the black step-like signal in (a) and of the AI measurements in (b). (d) Full signal measured by the hybrid Mas–AI sensor aboard the A300–0gaircraft during successive 1-gand 0-gphases of the flight. For this data set, where 2TMA=3 ms, SNR=4.3 andTc=500 ms, the resolution of the sensor in one second is more than 100 times below the plane acceleration fluctuationsδam. Figure 3a–c illustrate the measurement process that we use to measure the plane acceleration during successive 1 g and 0 g phases of the flight ( Fig. 3d ), with high resolution. Figure 3: High resolution measurement of the plane acceleration. ( a ) In red, signal recorded by the MAs in the time window (−2 T, 2 T ) around the measurement times t i = iT c (vertical green lines), with T c =500 ms and 2 T =3 ms. The MAs signal has been filtered by the response function of the AI described in the Methods section, and the red points represent the value of the signal at t i . This value determines the reciprocity region where the AI operates, delimited by two horizontal dashed lines. In this way, the MAs provide the coarse acceleration measurement (black step-like signal). ( b ) The AI is then used for the high-resolution measurement within its reciprocity region, bounded by the two blue dashed lines at ± a R /2, with a R = π / kT 2 ≈0.087 m s −2 . The error bars represent the noise of the atom accelerometer, which equals 0.0065 m s −2 per shot in this example (SNR=4.3). ( c ) The total acceleration ( a m ) is the sum of the black step-like signal in ( a ) and of the AI measurements in ( b ). ( d ) Full signal measured by the hybrid Mas–AI sensor aboard the A300–0 g aircraft during successive 1- g and 0- g phases of the flight. For this data set, where 2 T MA =3 ms, SNR=4.3 and T c =500 ms, the resolution of the sensor in one second is more than 100 times below the plane acceleration fluctuations δa m . Full size image Main error sources Because of their limited performances, mainly their nonlinear response and intrinsic noise (Methods), the MAs provide a signal that is not perfectly proportional to the acceleration a m . This leads to errors on the estimated acceleration a E that blur the MAs–AI correlation function and might prevent from finding the fringe index n ( t i ) where the AI operates. These errors increase with the AI sensitivity and with the acceleration signal a m . For a given acceleration level, the good measurement strategy consists in increasing T up to T MA where the MAs can still resolve the correlation fringes. This will set the scale factor of the AI. The sensitivity of the accelerometer is then determined by the SNR of the matter-wave sensor, which is estimated independently from the MAs with our method. For instance at 1 g , where δa m ∼ 0.5 m s −2 , the MAs enables us to increase the AI interrogation time up to 2 T MA =6 ms and to resolve the correlation fringes. Future improvements will rely on the use of well-characterized MAs, in particular on a calibration of their scale factor at the 10 −3 level over the sensitivity bandwidth of the AI, to achieve interrogation times 2 T MA >20 ms. High-frequency (>10 Hz) vibration damping could also be used to constrain the frequency range where the MAs are needed, and, therefore, push forward a particular sensor technology. Second, parasitic inertial effects due to the rotation of the plane might be experienced by the matter-wave sensor and not by the MAs. At 1 g , the atoms fall down before interacting with the Raman beams (aligned along the Y axis), so that the interferometer has a physical area and is thus sensitive to the Sagnac effect. The resulting Coriolis acceleration, measured by the AI and not by the MAs, might impair the correlation and limit the performance of the hybrid sensor. For shot-to-shot fluctuations of the plane rotation of the order of 10 −3 rad s −1 , we estimate a limit to the sensitivity at the 10 −4 m s −2 level at 1 g . This error source may be significantly reduced in the future with the use of extra sensors to measure the rotation of the plane and to take it into account in the calculation of the estimated acceleration. Finally, the atomic SNR limits the sensitivity of the inertial sensor. During the flight, we measure at 1 g a SNR of 3.1 for 2 T =6 ms, which is in agreement with the value measured in our laboratory for the same interrogation time. With our experimental setup, the signal ( A ∼ 0.1) is essentially limited by the imperfections of the atomic beam splitters and mirror due to the temperature of the cloud and to the gaussian intensity profile of the Raman beams, whereas the noise is mainly due to detection noise. In these conditions, with Tc =500 ms, the acceleration noise of the AI equals . At this sensitivity level, the hybrid sensor is able to measure inertial effects more than 300 times weaker than the typical acceleration fluctuations of the aircraft. We emphasize that reaching such a high resolution is possible because of the appropriate combination of MAs (Methods), the success of operating the AI in the plane, and the use of our method for the acceleration measurement. In the present configuration of the experiment, the SNR degrades at 1 g when 2 T increases above 20 ms because the atoms fall down and escape the Raman and detection beams [12] . This limitation could be overcome because of extra Raman beam collimators and by changing the orientation of the detection lasers. In 0 g , the experiment falls with the atoms and the SNR is not constrained by gravity any more. The SNR may also be improved significantly in the future because of a better detection system (for example, more stable detection lasers) and the use of ultra-cold atoms. Differential measurement in 0 g We focus now on the microgravity operation of the matter-wave inertial sensor and on its possible application to fundamental physics tests such as that of the UFF. Such a test can be carried out with two AIs measuring the acceleration of two different atoms with respect to the same mirror that retroreflects the Raman lasers. In airborne or spaceborne experiments, the mirror constitutes an ill-defined inertial reference because of the craft's vibrations. This might degrade the sensitivity of the test, unless the vibrations impact the two interferometers in the same way. Vibration noise rejection occurs when conducting differential measurements such as in the operation of gradiometers [25] or gyroscopes [26] , and is expected in UFF tests based on atom interferometry [16] . The rejection efficiency depends on the two species used for the UFF test and is maximum for simultaneous interrogation of the two atoms ( Supplementary Information ). In the case of a finite rejection, the impact of the acceleration noise can further be reduced by measuring the vibrations of the mirror with MAs to substract them from the differential phase measurement. In this way, the MAs are used to release the requirements on the vibration damping of the craft as they measure the accelerations not rejected in the differential operation of the two AIs. The efficiency of that technique is limited by the performances of the MAs as their imperfections (for example, their nonlinearities) translate into residual vibration noise impairing the differential acceleration measurement. In the following, we investigate vibration noise rejection by operating our 87 Rb sensor in a differential mode. We use a sequence of four light pulses to build a two-loop AI [25] that is equivalent to two successive one-loop interferometers head to tail ( Fig. 4b ). The four-pulse AI provides a signal resulting from the coherent substraction of two spatially and temporally separated inertial measurements and is therefore expected to be less sensitive to the low-frequency inertial effects. 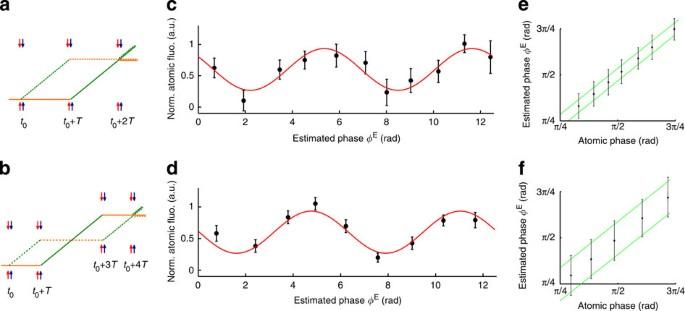Figure 4: Comparison of two AI geometries in 0g. (a,b) 3-pulse and four-pulse interferometers considered in this work. (c,d) Corresponding MAs–AI correlation functions recorded during the 0gphase of consecutive parabolas, with total interrogation times of 2T=20 ms and 4T=20 ms, respectively. To obtain these plots, we have sorted the estimated phase data (200 and 180 points, respectively) and averaged the correlation points by packets of 20. The error bars equal the standard deviation of each packet divided by, and are transferred to the vertical axis in this averaging procedure. The red line is a sinusoidal fit to the points. To make the comparison of the two correlations easier, we have scaled the vertical axis so as to obtain the same amplitude for the two sinusoids. (e,f) Comparison of the total correlation noiseσcorr(error bars) and of the atomic phase noisefor the two interferometer geometries (the vertical spacing between the green lines is 2σAI). The atomic phase data {Φ(ti)} have been obtained from the atomic measurements {P(ti)} by inverting the AI modelPAI(Φ), in the linear region of the interferometer ranging fromΦ≈π/4 toΦ≈3π/4. To facilitate the comparison ofσcorrandσAI, we have setΦE=Φ(the points are thus aligned on the first bisector). Figure (e) (resp. (f)) shows that the sensitivity of the sensor is limited by the vibration noiseσvibnot measured by the MAs (respectively by the atomic phase noise). Figure 4: Comparison of two AI geometries in 0 g . ( a , b ) 3-pulse and four-pulse interferometers considered in this work. ( c , d ) Corresponding MAs–AI correlation functions recorded during the 0 g phase of consecutive parabolas, with total interrogation times of 2 T =20 ms and 4 T =20 ms, respectively. To obtain these plots, we have sorted the estimated phase data (200 and 180 points, respectively) and averaged the correlation points by packets of 20. The error bars equal the standard deviation of each packet divided by , and are transferred to the vertical axis in this averaging procedure. The red line is a sinusoidal fit to the points. To make the comparison of the two correlations easier, we have scaled the vertical axis so as to obtain the same amplitude for the two sinusoids. ( e , f ) Comparison of the total correlation noise σ corr (error bars) and of the atomic phase noise for the two interferometer geometries (the vertical spacing between the green lines is 2 σ AI ). The atomic phase data { Φ ( t i )} have been obtained from the atomic measurements { P ( t i )} by inverting the AI model P AI ( Φ ), in the linear region of the interferometer ranging from Φ ≈ π /4 to Φ ≈3 π /4. To facilitate the comparison of σ corr and σ AI , we have set Φ E = Φ (the points are thus aligned on the first bisector). Figure ( e ) (resp. ( f )) shows that the sensitivity of the sensor is limited by the vibration noise σ vib not measured by the MAs (respectively by the atomic phase noise). Full size image To illustrate the noise rejection, we operate the three-pulse and four-pulse interferometers with a same total interrogation time of 20 ms, and compare the MAs–AI correlation for each geometry ( Fig. 4 ). Figure 4c,d show that the quality of the correlation (ratio of the sinusoid contrast to the mean error bar) is clearly improved in the differential geometry compared with the 3-pulse interferometer. To understand this difference, we estimate the total noise of the correlation, defined as . It results, in the linear range of the interferometer, from the quadratic sum of two independent contributions: the atomic phase noise , and the vibration noise σ vib not measured by the MAs. As we can estimate σ AI independently from the correlation (see the second subsection in Methods), the comparison of σ corr and σ AI indicates whether the sensor sensitivity is limited by the atomic noise ( σ corr ≈ σ AI ) or by the residual vibration noise ( σ corr > σ AI ). In Figure 4e,f , we have represented σ corr (error bars) and σ AI (vertical spacing between the green lines) for the one-loop and the two-loop interferometers, respectively. Figure 4e shows that the sensitivity of the three-pulse sensor is limited by the vibration noise not measured by the MAs, as σ corr > σ AI . On the contrary, Figure 4f reveals that the atomic phase noise is the main limit to the sensitivity of the four-pulse sensor, as σ corr ≈ σ AI . The SNR in the four-pulse interferometer is less than in its three-pulse counterpart as the extra light pulse reduces the interference fringe contrast due to the Raman beam intensity inhomogeneities and the transverse temperature of the cloud. In spite of greater atomic noise, the quality of the correlation 4f is better than that of correlation 4e, which shows that the four-pulse sensor operates a vibration noise rejection. In the four-pulse geometry, the two elementary interferometers operate one after another and share accelerations of frequency below 1/2 T . In a UFF test, two AIs of equal scale factor ( kT 2 ) will interrogate two different atoms almost simultaneously, so that the noise rejection is expected to be much more efficient (see ref. 16 and Supplementary Information ). In that case, the precision of the inertial sensor might be limited by the atomic phase noise, that is, by the SNR of the interferometer. For the 3-pulse AI data in Figure 4c, e (2 T =20 ms), we estimate a SNR of 2.1, which corresponds to an acceleration sensitivity of the matter-wave sensor of , in the context of the high-vibration noise rejection expected for the UFF test. That sensitivity level may be greatly improved in the future by using a highly collimated atomic source in microgravity [13] . We finally discuss possible improvements of our setup, both for inertial guidance and fundamental physics applications. In the former case, increasing the resolution of the accelerometer will be achieved by using well-characterized MAs to increase T MA , and by improving the SNR of the AI. Reaching an interrogation time 2 T MA =40 ms in the plane (where the acceleration fluctuations are δa m ∼ 0.5 m s −2 r.m.s. at 1 g ) would require MAs whose scale factor frequency response is determined with a relative accuracy of 2×10 −4 . We believe that such precision can be achieved with state-of-the-art MA technology, for example, capacitive MicroElectroMechanical Systems (MEMS) sensors, and we now work at implementing these sensors in our setup. Together with a shot noise limited AI with SNR ∼ 200 (as in ref. 26 ), the resolution of the hybrid sensor would be 8×10 −7 m s −2 per shot, which would represent a major advance in inertial navigation as well as in airborne gravimetry. We note that the present analysis does not report the in-flight bias of the matter-wave sensor because no other airborne accelerometer of similar accuracy was available onboard to proceed to the comparison. However, it has been demonstrated in laboratories that atom accelerometers can reach biases of the order of 10 −8 m s −2 under appropriate conditions [27] . Tests of fundamental physics would also require performant MAs to remove the residual aircraft's or satellite's acceleration noise not rejected in the differential measurement. For a UFF test in the 0 g plane and a vibration rejection efficiency of 300 (explained in ref. 16 and in the Supplementary Information ), a differential acceleration sensitivity of 3×10 −10 m s −2 per shot (SNR=200, 2 T =2 s) could be achieved with MAs of 2×10 −4 relative accuracy, if the vibrations during the 0 g phase are damped to the 5×10 −4 m s −2 level. In space, high-performance MAs such as the sensors developed for the GOCE mission could be used to determine the residual accelerations of the satellite ( ∼ 10 −6 m s −2 ) with a resolution [28] of the order of 10 −12 m s −2 . The vibration rejection efficiency of 300 would thus limit the impact of the acceleration noise on the interferometric measurement to 3×10 −15 m s −2 per shot, which would stand for a minor contribution in the error budget. Therefore, high-precision test of the equivalence principle could be conducted in space without the strong drag-free constraints on the satellite that represent a major challenge in current space mission proposals. To conclude, we have demonstrated the first airborne operation of a cold-atom inertial sensor, both at 1 g and in microgravity. We have shown how the matter-wave sensor can measure the craft acceleration with high resolutions. Our approach proposes to use mechanical devices that probe the coarse inertial effects and allow us to enter the fine measurement regime provided by the atom accelerometer. In the future, instruments based on the combination of better characterized mechanical sensors and a shot noise limited AI could reach sensitivities of the order of few 10 −7 m s −2 in one second aboard aircrafts. Thus, our investigations indicate that sensors relying on cold-atom technology may be able to detect inertial effects with resolutions unreached so far by instruments aboard moving crafts characterized by high acceleration levels. Cold-atom sensors offer new perspectives in inertial navigation because of their long-term stability as they could be used to correct the bias ( ∼ few 10 −5 m s −2 ) of the traditional sensors monitoring the crafts' motion, below the 10 −7 m s −2 level. In geophysics, airborne gravity surveys may also benefit from the accuracy of AIs [29] . Moreover, we have operated the first matter-wave sensor in microgravity. We have shown how differential interferometer geometries enable to reject vibration noise of the experimental platform where new types of fundamental physics tests will be carried out. Our result in 0 g suggests that the high sensitivity level of matter-wave interferometers may be reached on such platforms, and support the promising future of AIs to test fundamental physics laws aboard aircrafts, sounding rockets or satellites where long interrogation times can be achieved [17] . While many quantum gravity theories predict violations of the UFF, AIs may investigate its validity at the atomic scale, with accuracies comparable to those of ongoing or future experiments monitoring macroscopic or astronomical bodies [30] . AI response function and MAs–AI correlation For a time-varying acceleration a ( t ) of the retroreflecting mirror, the phase of the interferometer at time t i = iT c is given by where f is the acceleration response of the 3-pulse AI. It is a triangle-like function [16] that reads: with being the time of the first Raman pulse at the i th measurement. The mean acceleration that we infer is defined as a m = Φ / kT 2 . Because of the MAs, we estimate the phase Φ E ( t i ) which is expected to be measured by the interferometer by averaging in the time domain, the signal a MA ( t ) by the AI response function: The MAs–AI correlation function can be written as and expresses the probability to measure the atomic signal P ( t i ) at time t i , given the acceleration signal a MA ( t ) recorded by the MAs. The estimated acceleration used in Figure 2 is defined by a E = Φ E / kT 2 . For simplicity, we have neglected, in equation (1), the Raman pulse duration τ =20 μs with respect to the interrogation time 2 T. The exact formula can be found in ref. 31 and has been used in the data analysis to estimate the phase Φ E . Estimation of the AI response and signal to noise ratio We calculate the probability density function (PDF) of the AI measurements P ( t i ) and fit it with the PDF of a pure sine (a 'twin-horned' distribution) convolved with a gaussian of standard deviation σ P . The fit function reads: where N is a normalization factor. In this way, we estimate the amplitude A and the offset value P 0 of the interference fringes, that is, we estimate the AI response P AI ( Φ )= P 0 − A cos Φ . The fitted parameters A and σ P provide an estimate of the in-flight signal-to-noise ratio of the interferometer, given by SNR= A / σ P . 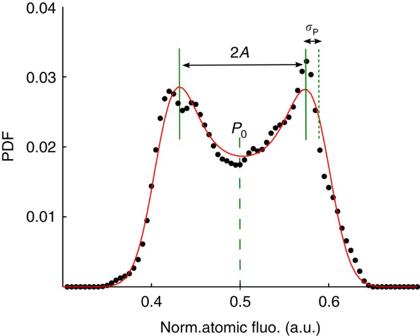Figure 5: Estimation of the AI response and SNR. PDF of the AI measurementsP(ti) (normalized atomic fluorescence) for the data ofFigures 2and3.P0andAare, respectively, the offset and the amplitude of the interference fringes, andσPis the standard deviation of the atomic noise. Figure 5 illustrates the method for the data used in Figures 2 , 3 , corresponding to the interrogation time 2 T =3 ms. The fitted parameters are P 0 =0.50, A =0.074 and SNR=4.3. Figure 5: Estimation of the AI response and SNR. PDF of the AI measurements P ( t i ) (normalized atomic fluorescence) for the data of Figures 2 and 3 . P 0 and A are, respectively, the offset and the amplitude of the interference fringes, and σ P is the standard deviation of the atomic noise. Full size image This method is independent on the MAs signal and informs both on the response of the AI, and on its one-shot acceleration sensitivity σ a =1/(SNR× kT 2 ). The characteristics of the interferometer are thus known without any extra calibration procedure. In particular, we can estimate the noise level of the matter-wave sensor, given by for a white atomic phase noise, and which equals for the data in Figure 5 , where T c =500 ms. Our analysis estimates the SNR by taking into account only the atomic noise due to detection noise or fluctuations of the fringe offset and contrast. It does not account for the laser phase noise that could impact the sensitivity of the acceleration measurement for long interrogation times [32] . However, we demonstrated the low phase noise of our laser system during previous parabolic flight campaigns [12] , which is at least one order of magnitude below the estimated atomic phase noise for the interrogation times we consider in this work ( T ≤10 ms). Therefore, we have neglected in this communication the laser phase noise contribution when evaluating the sensitivity of the sensor. Determination of the acceleration signal Because of the MAs signal, we first determine the fringe number n(t i )=floor[ a E ( t i )/ a R ] where the interferometer operates at time t i = i T c , with a R = π / kT 2 being the reciprocity interval of the matter-wave sensor. The values n ( t i ) are represented by the black step-like curve in Figure 3a . 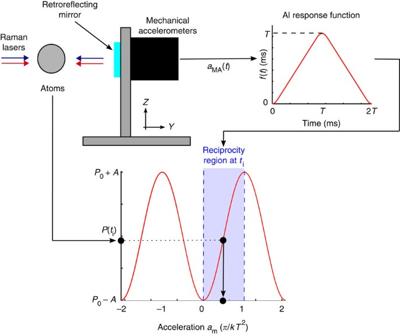Figure 6: Schematic of the two-step acceleration measurement process. The signal of the MAs is filtered by the response functionf(t) of the AI (described in the first paragraph of the Methods section) and informs on the reciprocity region where the AI operates at the measurement timeti=iTc. In this example, the reciprocity region corresponds to the 0−π/kT2interval, that is, ton(ti)=0. The value provided by the AI,P(ti), is then used to refine the acceleration measurement within the reciprocity region. The accelerationis obtained fromP(ti) by inverting the AI responsePAI(am) (red curve). Second, we use the atomic measurements P ( t i ) to deduce the acceleration measured by the AI in its reciprocity region [ n ( t i ) a R , ( n ( t i )+1) a R ], and given by: The total acceleration is finally computed as: The acceleration measurement process is illustrated in Figure 6 . Figure 6: Schematic of the two-step acceleration measurement process. The signal of the MAs is filtered by the response function f ( t ) of the AI (described in the first paragraph of the Methods section) and informs on the reciprocity region where the AI operates at the measurement time t i = iT c . In this example, the reciprocity region corresponds to the 0− π /k T 2 interval, that is, to n ( t i )=0. The value provided by the AI, P ( t i ), is then used to refine the acceleration measurement within the reciprocity region. The acceleration is obtained from P ( t i ) by inverting the AI response P AI ( a m ) (red curve). Full size image Limitations due to the Mechanical Accelerometers The main limitation of the MAs comes from the nonlinearities in their frequency response (phase and gain), which means that the signal a MA ( t ) is not exactly proportional to the acceleration of the retroreflecting mirror. This results in errors in the estimation of the phase Φ E that impair the MAs–AI correlation. The nonlinearities typically reach amplitudes ɛ nl ∼ 5% within the AI bandwidth that equals 1/2 T ≤500 Hz. (The acceleration frequency response H ( ω ) of an AI has been measured in ref. 33 and corresponds to the response of a second-order low pass filter of cut-off frequency 1/2 T ). To reduce them, we combine two mechanical devices of relatively flat frequency response within two complementary frequency bands: a capacitive accelerometer (Sensorex SX46020) sensing the low-frequency accelerations (0–1 Hz), and a piezoelectric sensor (IMI 626A03) measuring the rapid fluctuations (1–500 Hz). In this way, we achieve ɛ nl ∼ 2%. For 2 T MA =6 ms, these nonlinearities correspond to errors on Φ E of about 0.5 rad r.m.s. Further details on the errors in the estimation of the phase due to the MAs nonlinearities are given in the Supplementary Information . Another limitation comes from the MAs internal noise, especially that of the capacitive one whose noise level integrated in (0–1 Hz) equals 3×10 −4 m s −2 . This noise is about one order of magnitude lower than this due to the nonlinearities of the MAs, and is independent of the acceleration level in the plane. Axis cross-talk of the MAs of the order of 2% is taken into account for the estimation of the phase, so that the errors on Φ E due to the MAs-axis coupling are negligible. Finally, the bias of the capacitive accelerometer is specified at the 0.05 m s −2 level, so that the mean estimated acceleration might drift during the flight (4 h). This results in a displacement of the dark-fringe position in the MAs–AI correlation plots. How to cite this article: Geiger, R. et al . Detecting inertial effects with airborne matter-wave interferometry. Nat. Commun. 2:474 doi: 10.1038/ncomms1479 (2011).